Ultrahigh-speed rotating nanoelectromechanical system devices assembled from nanoscale building blocks The development of rotary nanomotors is crucial for advancing nanoelectromechanical system technology. In this work, we report design, assembly and rotation of ordered arrays of nanomotors. The nanomotors are bottom-up assembled from nanoscale building blocks with nanowires as rotors, patterned nanomagnets as bearings and quadrupole microelectrodes as stators. Arrays of nanomotors rotate with controlled angle, speed (over 18,000 r.p.m. ), and chirality by electric fields. Using analytical modelling, we reveal the fundamental nanoscale electrical, mechanical and magnetic interactions in the nanomotor system, which excellently agrees with experimental results and provides critical understanding for designing metallic nanoelectromechanical systems. The nanomotors can be continuously rotated for 15 h over 240,000 cycles. They are applied for controlled biochemical release and demonstrate releasing rate of biochemicals on nanoparticles that can be precisely tuned by mechanical rotations. The innovations reported in this research, from concept, design and actuation to application, are relevant to nanoelectromechanical system, nanomedicine, microfluidics and lab-on-a-chip architectures. Nanoelectromechanical system (NEMS) devices, consisting of both electronic and mechanical components, are emerging as the next-generation technology that can significantly impact people’s lives. It has intrigued the research community for over a decade, not only because of the rich fundamental science where devices are made on the nanoscale [1] but also because of the high potential of making technical breakthroughs in various areas including robotics [2] , biomedical research [3] , [4] , [5] , [6] , and optoelectronics [7] . Rotary nanomotors, a type of NEMS devices, are particularly critical for advancing NEMS technology in converting electric energy into nanoscale mechanical motions for nanomachines and nanofactories [8] , [9] . Traditional fabrication of miniature motors requires complex design and arduous processes [10] , [11] , [12] , [13] . For instance, a simple rotary microelectromechanical system (MEMS) device requires fabrication and integration of multiple components including rotors, bearings, hubs and stators all on miniaturized scales [9] , [10] , [11] , [14] . Using traditional MEMS technologies—photolithography and micromachining—borrowed from the microelectronics industry, hundreds of fabrication steps are required. The devices suffer from low yield and short lifetime [15] . Only several rotary MEMS were made on each wafer and most of them just operated from a few seconds to a few hours [10] , [16] . Therefore, it is extremely difficult to apply techniques learned in MEMS to the fabrication of even smaller NEMS devices. This is also evidenced by the restricted sizes of MEMS motors of millimetres to hundreds of micrometres [16] , [17] , [18] . Few can reach tens of micrometres and very few can make truly nanoscale motors even using the best available techniques [12] , [13] , [19] . It is highly desirable to investigate new mechanisms to realize large arrays of rotary NEMS devices with high efficiency, nanoscale dimensions, reliable performance and at a low cost. Recently, intensive research efforts have been focused on using nanoentities as actuation components for MEMS/NEMS devices owing to the unique advantages provided by nanotechnology: (1) large arrays of nanoentities with controlled geometry, chemical, physical and mechanical properties can be routinely synthesized at low cost [20] ; (2) The size of the MEMS devices can be significantly shrunk by using synthesized nanoentities as building blocks [1] ; and (3) The unique physical/chemical/electrical properties of nanoparticles improve the performance of miniaturized mechanical devices [21] , [22] . A group at UC Berkeley fabricated nanomotors with top-down multistep electron beam lithography [12] . In such a device, a nanoscale metal pad was attached to a piece of suspended multiwall carbon nanotube via electron beam lithography. With high electric voltages, the metal pad rotated around the multiwall carbon nanotube with the inner walls of carbon nanotubes serving as bearings. The excellent demonstration of nanoentities for rotary NEMS, however, required complex fabrication procedure. Recently, a group at Cornell University made another type of nanomotors based on inorganic and organic hybrid structures [13] . Molecular motors, a type of rotary protein, were used as the driving component of the nanomotors. Lithographically patterned inorganic nanorods attached to the molecular motors were used as rotors. When hydrolysing adenosine triphosphate, the molecular motors can make the inorganic nanorods rotate. Owing to the complexity of the conjugation of inorganic nanorods to molecular motors, only a few nanorods out of hundreds had been rotated. Also, limited by the characteristics of natural molecular motors, the devices could not alter either their rotation or speed. Catalytic nanomotors have emerged as a new type of nanomechanical devices that convert chemical energy to mechanical motions [8] , [23] , [24] . Most of the catalytic motors have been actuated to transport biomolecules, such as proteins or bacteria [25] . Recently, it was demonstrated that asymmetrical and one-end fixed nanorods could rotate [26] , [27] , nevertheless, with random speed, orientation and locations. In this work, we report innovative design and mechanisms for assembling and operating arrays of rotary NEMS devices made from nanoscale building blocks. The nanomotors consist of multisegment nanowires, patterned nanomagnets and quadrupole microelectrodes as rotors, bearings and stators, respectively. Arrays of nanomotors can be assembled and rotated with controlled angle, speed (to at least 18,000 r.p.m.) and chirality. The fundamental electric, magnetic and mechanical interactions involved in the components of the nanomotor systems were investigated that provide understanding for designing and actuating various metallic NEMS devices. The nanomotors, with all the dimensions <1 μm, can robustly rotate for 15 h for >240,000 cycles and were demonstrated for controllable biochemical release. The innovation in this research may inspire multiple research fields including MEMS/NEMS, bio-NEMS, micro/nanofluidics and lab-on-a-chip architecture. Design of nanomotors We investigated a unique type of nanomotors made of strategically assembled nanoentities, such as nanowires and nanodisks, as shown in Fig. 1a,b . The nanomotors consist of multisegment Au/Ni/Au nanowires (150–400 nm in diameter and ~800 nm to 10 μm in length) acting as rotors, patterned nanomagnets (200 nm to 2 μm in diameter) acting as bearings and simple quadruple microelectrodes acting as stators. The patterned nanomagnets are the core components for the anchorage of the rotary parts. The nanomagnets consist of tri-layer thin-film stacks of Au/M/Cr, where M represents magnetic materials such as Ni and Co. Each layer in the nanomagnets serves a purpose as follows: the bottom Cr layer adheres to the substrate, the middle magnetic layer provides the magnetic field and the top Au layer is used for adjusting the spacing between the magnetic layer and the nanowires in order to tune the magnetic attraction. The magnetic attraction can be adjusted so precisely that it can anchor the nanowires to the bearings, but not too tightly to prevent the nanowires from rotating. 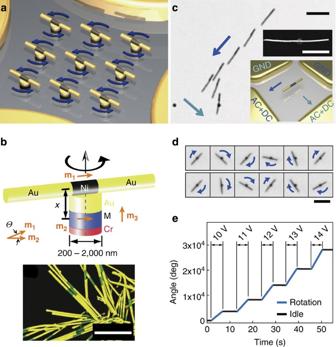Figure 1: Design, assembly and actuation of nanomotors. (a) Schematic diagram of an array of nanomotors assembled from nanoscale building blocks with multisegment Au/Ni/Au nanowires as rotators, tri-layer Au/Ni/Cr magnets as bearings and microelectrodes as stators. (b) Schematic diagram of a nanomotor and a SEM image of Au/Ni/Au nanowires highlighted in false colours (yellow: Au; green: Ni). Scale bar, 5 μm. (c) Overlapped images of an Au/Ni/Au nanowire transported and assembled on a nanobearing by the electric tweezers. Scale bar, 10 μm. (Inset) SEM image of an assembled nanomotor (scale bar, 5 μm) and a schematic diagram of electric tweezers manipulating a nanowire. (d) Snapshots of a nanowire rotating on a nanobearing CW and CCW every 71 ms. Scale bar, 10 μm. (e) Angular positionθof an assembled nanowire in ACE-fields of 10–14 V (rotor: Au (4.5 μm)/Ni (1 μm)/Au (4.5 μm); bearing: a thin-film stack made of Au (100 nm)/Ni (80 nm)/Cr (6 nm) and 1 μm in diameter). Figure 1: Design, assembly and actuation of nanomotors. ( a ) Schematic diagram of an array of nanomotors assembled from nanoscale building blocks with multisegment Au/Ni/Au nanowires as rotators, tri-layer Au/Ni/Cr magnets as bearings and microelectrodes as stators. ( b ) Schematic diagram of a nanomotor and a SEM image of Au/Ni/Au nanowires highlighted in false colours (yellow: Au; green: Ni). Scale bar, 5 μm. ( c ) Overlapped images of an Au/Ni/Au nanowire transported and assembled on a nanobearing by the electric tweezers. Scale bar, 10 μm. (Inset) SEM image of an assembled nanomotor (scale bar, 5 μm) and a schematic diagram of electric tweezers manipulating a nanowire. ( d ) Snapshots of a nanowire rotating on a nanobearing CW and CCW every 71 ms. Scale bar, 10 μm. ( e ) Angular position θ of an assembled nanowire in AC E -fields of 10–14 V (rotor: Au (4.5 μm)/Ni (1 μm)/Au (4.5 μm); bearing: a thin-film stack made of Au (100 nm)/Ni (80 nm)/Cr (6 nm) and 1 μm in diameter). Full size image Assembling and actuation of nanomotors To realize such nanomotors, there are two fundamental problems to be addressed such as (1) how to precisely assemble nanomotors with nanowires anchoring on the patterned nanomagnets? and (2) how to rotate the nanomotors? Here we exploited the use of ‘electric tweezers’ to resolve these problems. Electric tweezers are our recently invented nanomanipulation technique that can transport nanoentities, such as nanowires and nanotubes, along arbitrary trajectories to designated positions with a precision of 150 nm [28] , [29] , [30] and rotate them with prescribed angle, speed and chirality [31] . The nanowire rotors, vital components of the rotrary nanomotors, were designed with a three-segment Au/Ni/Au structure, where the Ni segment serves to anchor the nanowires on the patterned magnetic bearings. Here, Au/Ni/Au nanowires were fabricated by electrodeposition into nanoporous templates in a three-electrode cell setup as detailed in the experimental session [28] , [32] . Nanowire suspension (4 μl) in deionized (DI) water was introduced into a reservoir of volume of ~4 μl that was made of polydimethylsiloxane elastomers assembled on top of the microelectrodes. Then the reservoir was sealed with a glass cover slip. By using electric tweezers, the nanowires can be transported by the DC E -field and aligned either parallel (AC//DC) or perpendicular (AC ⊥ DC) to their transport directions by the AC E -field. By controlling the durations of the combined AC and DC E -fields in both the X and Y directions, the nanowires can be precisely manipulated in two dimensions along prescribed trajectories to the patterned magnetic bearings as shown in Fig. 1c and Supplementary Movie 1 . When positioned in the vicinity of a nanobearing, the nanowire is swiftly attracted and assembled atop of the nanobearing by the magnetic force between the nanowire and nanobearing. Once anchored on the nanobearing, the nanowire cannot be moved by the E -fields any more. In such a manner, we can readily form ordered arrays of nanomotors by transporting and assembling nanowires in series. Owing to the efficient manipulation by the electric tweezers, each assembling event only takes a few seconds. The nanobearings (200 nm to 2 μm in diameter), anchoring nanowire rotors, have an embedded Ni film with a gently tilted perpendicular magnetic anisotropy to provide magnetic anchoring force ( Supplementary Fig. 1 and Supplementary Note 1 ) [33] . The in-plane magnetic orientation of the nanobearings is controlled by demagnetization with a gradually reducing oscillating magnetic field of ±10 kG followed by re-magnetization at 10 kG along a desired direction for 5 s. Applying four AC voltages (10–150 kHz and 8–17 V) with a sequential phase shift of 90° on the quadruple microelectrodes, we created a rotating AC E -field that can instantly drive arrays of nanowires to rotate atop of the magnetic bearings. The motions of the rotating nanomotors were captured by an optical microscope equipped with a CCD camera operating at 14–200 frames per second. The nanomotors were rotated both clockwise (CW) and counter CW (CCW), same as that of the rotating E -fields as shown in Fig. 1d . At each AC voltage, the rotation instantly started, reached a terminal velocity and stopped as soon as the external E -field was removed without observable acceleration or deceleration ( Fig. 1e ). The instant rotation response is because of the extremely low Reynolds number of 10 −5 for nanowires in DI water, where the viscous force overwhelms the motion [34] . Taking a closer look, we noticed that the plot of rotation angle ( θ ) versus time ( t ) was not completely linear ( Fig. 2a ). By taking the first derivative of angle with respect to time, we could obtain rotation speed ( ω ) that showed a clear sinusoidal dependence on time ( t ) and angle ( θ ) oscillating between two states such as the high speed ( ω max ) and the low speed states ( ω min ) with a periodicity of 360° ( Fig. 2b,c ). To understand these phenomena, a thorough investigation of electric, magnetic and mechanical forces/torques in the nanoscale components of a nanomotor system is highly desirable. 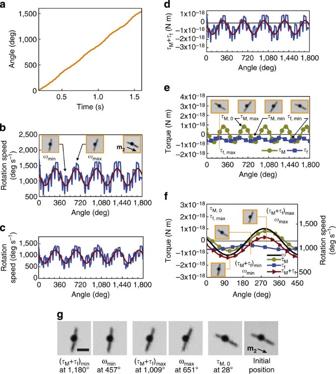Figure 2: Characteristics of rotational dynamics. (a) Rotation angle (θ) versus time (t). (b,c) Rotation speed (ω) versus angular position (θ) of the nanomotor at (b) 12 V; and (c) 11 V and 10 kHz (CW). (d) Sum of the magnetic (τM) and friction torques (τf): (τM+τf) exerted on the motor at 12 V and 10 kHz. (e) Analytical solutions ofτMandτfversus angle with the snapshots illustrating the angular position of the nanomotor forτM,0,τM,max,τM,min,τf,maxandτf,min. (f) Angle-dependent torques of (τM+τf),τM,τf, and rotation speedωof the nanorotor at 12 V and 10 kHz. The snapshots showed the angular positions of the nanomotor when the rotation speeds are the maximum (ωmax), minimum (ωmin), the combined magnetic and frictional torque of (τM+τf) is maximum, (τM+τf)minandτM,0, respectively. (g) The maximum/minimum rotation speeds of nanomotors occur when the combined torque of (τM+τf) is the maximum/minimum in the same direction ofE-field. The alignment of the rotating nanomotor atτM=0 is the same as the initial alignment of the just-assembled nanowire. Scale bar, 5 μm. Figure 2: Characteristics of rotational dynamics. ( a ) Rotation angle ( θ ) versus time ( t ). ( b , c ) Rotation speed ( ω ) versus angular position ( θ ) of the nanomotor at ( b ) 12 V; and ( c ) 11 V and 10 kHz (CW). ( d ) Sum of the magnetic ( τ M ) and friction torques ( τ f ): ( τ M + τ f ) exerted on the motor at 12 V and 10 kHz. ( e ) Analytical solutions of τ M and τ f versus angle with the snapshots illustrating the angular position of the nanomotor for τ M,0 , τ M,max , τ M,min , τ f,max and τ f,min . ( f ) Angle-dependent torques of ( τ M + τ f ), τ M , τ f , and rotation speed ω of the nanorotor at 12 V and 10 kHz. The snapshots showed the angular positions of the nanomotor when the rotation speeds are the maximum ( ω max) , minimum ( ω min ), the combined magnetic and frictional torque of ( τ M + τ f ) is maximum, ( τ M + τ f ) min and τ M,0 , respectively. ( g ) The maximum/minimum rotation speeds of nanomotors occur when the combined torque of ( τ M + τ f ) is the maximum/minimum in the same direction of E -field. The alignment of the rotating nanomotor at τ M =0 is the same as the initial alignment of the just-assembled nanowire. Scale bar, 5 μm. Full size image Nanoscale interactions in the nanomotors Five torques can be identified in the nanomotor system given by: where τ e , τ e ′, τ η , τ M , and τ f are the electric torque because of the rotating AC E -fields, effective torque because of the induced electric polarization of the nanowire and bearing, viscous drag torque from the water medium, magnetic and frictional torques between the magnetic segment of the nanowire and the magnetic nanobearing, respectively. The viscous drag torque τ η on a rotating nanowire in DI water is calculated as [35] : where r and l are the radius and length of the nanowire, respectively, η is the viscous coefficient of suspension medium and N is the number of nanowire segments used for estimation of the viscous drag torque, which is taken as 2. For a nanowire of 150 nm in radius and 10 μm in length, τ η = −1.74 × 10 −19 ω (N m). We note that in addition to the viscous drag torque discussed above, a nanowire rotating close to a substrate also experiences a wall effect, which is much smaller compared with other involved forces or torques and can be safely omitted ( Supplementary Note 2 ). The electric torque is generated by the interaction of the polarized nanoparticles with the AC E -fields, given by [36] where ε m and Im( K ) are the permittivity of the suspension medium and the imaginary part of the Clausius–Mossotti factor K of the nanowire, respectively, and E is the intensity of the E -field created by the applied voltage V ( E ∝ V ). As τ e solely depends on the suspension medium, Im( K ), and the dimension of a nanowire, the value of τ e for an assembled nanowire rotor should be identical with that for the same nanowire freely rotating in suspension. Note that for a free rotating nanowire, the electric torque balances with the viscous torque ( τ e = τ η ). Therefore, by combining equations (2) and (3), the electric torque ( τ e ) for the assembled nanowire rotor can be readily calculated from that of a free rotating nanowire, which reveals the rotation speed ω ∝ V 2 . Indeed, the linear dependence of ω versus V 2 was experimentally observed, with a slope of as shown in Fig. 3a (orange line, for the free rotating nanowire). Therefore, the electric torque can be readily determined as τ e =3.01 × 10 −20 V 2 (N m V −2 ]). At a given voltage, for example, 12 V, the nanowire rotor receives an electric torque of 4.33 pN μm. 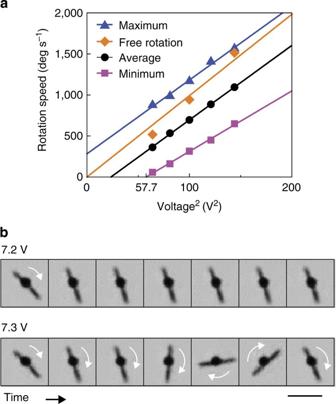Figure 3: Rotation speed at different voltages and the threshold voltage. (a) High (blue), low (magenta) and average (black) rotation speeds of a nanomotor (rotor: Au(4.5 μm)/Ni(1 μm)/Au(4.5 μm) nanowires, 2 μm diametered bearings made of a thin-film stack of Au(100 nm)/Ni (80 nm)/Cr (6 nm)) linearly increase withV2(the same was observed for nanomotors with bearings of 500 nm to 1 μm as in theSupplementary Fig. 4). For the same nanowire freely rotating in suspension, the rotation speeds increase withV2with a steeper slope (orange). (b) Snapshots of the nanomotor taken every 400 ms at AC voltages of 7.2 and 7.3 V show the that the threshold voltage is 7.3 V. Scale bar, 10 μm. Figure 3: Rotation speed at different voltages and the threshold voltage. ( a ) High (blue), low (magenta) and average (black) rotation speeds of a nanomotor (rotor: Au(4.5 μm)/Ni(1 μm)/Au(4.5 μm) nanowires, 2 μm diametered bearings made of a thin-film stack of Au(100 nm)/Ni (80 nm)/Cr (6 nm)) linearly increase with V 2 (the same was observed for nanomotors with bearings of 500 nm to 1 μm as in the Supplementary Fig. 4 ). For the same nanowire freely rotating in suspension, the rotation speeds increase with V 2 with a steeper slope (orange). ( b ) Snapshots of the nanomotor taken every 400 ms at AC voltages of 7.2 and 7.3 V show the that the threshold voltage is 7.3 V. Scale bar, 10 μm. Full size image The induced torque ( τ e′ ) because of the electrically polarized nanorotor and nanobearing in an external AC E -field has a much lower, though non-negligible, effect on the nanomotor than that of the driving electric torque ( τ e ). This induced torque has two roles on the rotation of nanomotors, both of which are proportional to E 2 and thus V 2 : first, it directly hinders the rotation of nanorotors; second, it results in an additional frictional torque between the rotor and bearing because of the electrostatic attraction, besides that arisen from the magnetic attraction. These two effects can be known from the slopes of ω – V 2 plots in Fig. 3a , where the rotation slopes of a nanowire motor (blue, black and magenta) are consistently lower than that of the same nanowires when freely rotating (orange). Note that no other torques, either the magnetic ( τ M ) or frictional torques ( τ f ), given in Equation (1) depends on the external E -fields. Therefore, the reduced slope is a sole result of the induced torques between the electrically polarized nanowire and bearing. Based on this understanding, we can calculate the induced torque as τ e′ = bV 2 , where b is a constant that equals to −2.52 × 10 −21 (N m V −2 ), from rotation of the free/anchored nanowire in Fig. 3a . The b value is ~1/10 of that for the electric torque ( τ e ), showing the non-negligible effect of the induced electric torques in components of metallic NEMS devices. Given the drag ( τ η ), electric ( τ e ) and induced torques owing to the polarization ( τ e′ ), the sum of the non- E -field dependent magnetic ( τ M ) and frictional torques ( τ f ) exerted on the nanowire rotors can be readily known from Equation (1). The combined torques of ( τ M + τ f ) exhibit a sinusoidal feature as shown in Fig. 2d , which counts for the angle-dependent periodic rotation of nanomotors in Fig. 2b,c ( Supplementary Fig. 2 ). To explicitly understand the contributions of the magnetic and frictional torques, we modelled the system using a simplified magnetic dipole–dipole interaction [37] . As shown in Fig. 1b , the angle-dependent magnetic torque between the rotor and bearing is determined by the horizontal magnetic moments of the nanowire ( m 1 ) and bearing ( m 2 ), given by τ ( x , Θ, m 1 , m 2 )= μ 0 ( m 1 m 2 sin Θ)/(4 πx 3 ), and the angle-dependent magnetic force is F ( x , Θ, m 1 , m 2 )=3 μ 0 ( m 1 m 2 cos Θ) (4 πx 4 )+ c , where μ 0 is the magnetic permittivity of vacuum, Θ is the angle between m 1 and m 2 , x is the separation distance between the nanowire and the Ni layer in the nanobearing, and the constant c is the magnetic force due to the magnetic moments of the nanobearing in the vertical direction ( m 3 ) and the horizontal magnetic moment of the nanowire ( m 1 ). If the friction coefficient at the interface of the nanowire and bearing is μ , the frictional torque τ f = μF , then ( τ M + τ f ) can be written as: where d , e and f are constants, θ and θ M are the angular positions of magnetic orientation of the nanowire and nanobearing, respectively, and Θ= θ − θ M . Fitting the experimentally obtained torque of ( τ M + τ f ) versus θ in Fig. 2d , we readily extracted the angular-dependent magnetic torque of τ M =−8.19 × 10 −19 sin(θ−27°) (N m) and frictional torque of τ f = −1.71 × 10 −19 cos(θ−27°) (N m) at 12 V and 10 kHz as shown in Fig. 2e . By using the same approach, the values of d , e , f and θ M were also determined for 10 and 11 V, which show excellent consistence with those obtained at 12 V ( Supplementary Note 3 and Supplementary Table 1 ). These results provide great support for our modelling, where the magnetic and its resulting frictional torque are independent of the applied E -field. We also note that the highest rotation speed ( ω max ) occurred neither when the magnetic torque has the highest value ( τ M,max ) in the same direction with the driving E -field, when the magnetic torque equals to zero ( τ M,0 ) aligning with the magnetic orientation of the bearing nor when the frictional torque has the lowest value ( τ f,min ). The highest/lowest speed occurred when the sum of ( τ M + τ f ) was maximum/minimum in the orientation of the electric torque (inset of Fig. 2f ). The feasibility of the modelling and torque analysis can be further confirmed by plotting the experimentally obtained highest ( ω max , blue) and lowest rotation speeds ( ω min , magenta) of the nanomotors at each applied voltage ( V ) as functions of V 2 ( Fig. 3a ). Both ω min and ω max linearly increase with V 2 , parallel to that of the average rotation speed ( ω AVG , black) versus V 2 , but vertically offset. Combining Equations (1)–(4), we obtained where δ =arctan ( e / d ). ω max and ω min occur when sin(θ−θ M + δ )=±1, respectively. The V 2 dependence in Equation (5) is consistent with the experimentally found V 2 dependence of ω min and ω max in Fig. 3a . The constant slope of ω–V 2 accounts for the parallel slopes of ω max – V 2 , ω min – V 2 and ω AVG – V 2 in Fig. 3a . Moreover, the x-intercept of ω min – V 2 can be used to estimate the threshold voltage ( V th ) required to initiate the rotation of nanomotors. It predicts a threshold voltage value of for a motor with a 2-μm-diameter bearing. This predicted value is very close to that of experimentally obtained 7.3 V, as the nanomotor failed to rotate a complete cycle up to 7.2 V ( Fig. 3b ). It indicates that the minimum required voltage to initiate the nanomotor rotation should overcome the maximum value of the combined magnetic and frictional torques ( τ M + τ f ) countering the electric torque. In summary, our modelling qualitatively revealed the distinct roles of various nanoscale torques involved in the nanomotor system, which excellently agreed with the experimental results. The new understandings from this investigation can be applied to design of various metallic NEMS devices. Ordered arrays of nanomotors To practically use the nanomotors for applications, it is important to evaluate the controllability, robustness and efficiency in assembling and rotating arrays of nanomotors. We patterned and rotated ordered 2 × 2 and 1 × 3 arrays of nanowire motors as shown in Fig. 4a,b and Supplementary Movies 2 and 3 . The manipulation and assembling of nanomotors do not require advanced skills, as the system is interfaced by user-friendly software. It took only ~10 s for a user, for example, a K-12 student, to assemble one motor after training and practicing for several times. It generally took <1 min to assemble a 2 × 2 array. Although the assembling efficiency is already much higher than those made by traditional lithographical techniques, which require advanced skills, training and education, we are in the process of developing an intelligent system to automate the nanowire recognition and manipulation for further improving the assembling efficiency of nanomotors. All nanomotors in the array started, stopped and reversed rotation simultaneously. The speed and chirality were precisely controlled by the voltages and phase shifts of the applied AC E -field ( Fig. 4c ). The rotation speeds of individual nanomotors were slightly different, which is because of the variations of dimensions of individual nanowires and bearings as well as their interfaces. 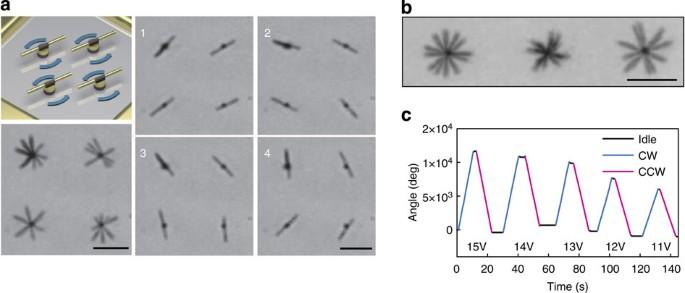Figure 4: Nanomotors assembled in ordered arrays. (a) Schematic diagrams and snapshot images of a 2 × 2 nanomotor array rotating CW at 12 V and 10 kHz. (b) Overlapped snapshot image of a 1 × 3 nanomotor array at 15 V and 10 kHz. Scale bars, 10 μm. (c) The rotation speed of nanomotors can be precisely controlled by ACE-fields as shown by rotation angle (θ) versus time at 15–11 V and 10 kHz. The nanomotors can instantly rotate in orientations both CW (blue) and CCW (magenta) and stop on demand. Figure 4: Nanomotors assembled in ordered arrays. ( a ) Schematic diagrams and snapshot images of a 2 × 2 nanomotor array rotating CW at 12 V and 10 kHz. ( b ) Overlapped snapshot image of a 1 × 3 nanomotor array at 15 V and 10 kHz. Scale bars, 10 μm. ( c ) The rotation speed of nanomotors can be precisely controlled by AC E -fields as shown by rotation angle ( θ ) versus time at 15–11 V and 10 kHz. The nanomotors can instantly rotate in orientations both CW (blue) and CCW (magenta) and stop on demand. Full size image Ultrahigh-speed rotation of nanomotors How fast can the nanomotors ultimately rotate? To test the limit, we optimized the AC E -field intensity and frequency. As aforediscussed, the rotation speed of nanomotors increases with E 2 . Simply narrowing the gap distance of the quadrupole electrodes from 500 to 100 μm, we readily increased E 2 by 625 times. The rotation speed also depends on the applied AC frequency. For 10 μm Au/Ni/Au nanowires in DI water, the maximum rotation speed was obtained experimentally at an E -field of 30 kHz ( Supplementary Fig. 3 ). Applying these optimized conditions, we rotated nanomotors to a speed of at least 18,000 r.p.m. at 17 V as shown in Supplementary Movie 4 (1,200 frames per second) and the Fig. 5a(inset) . The rotation orientation was CW as determined from the slowed motion in Supplementary Movie 5 (14 V). Agreeing with our other results, the rotation speeds (to at least 18,000 r.p.m.) were proportional to E 2 or V 2 , which counts for the ultrahigh-speed rotation at only 17 V ( Fig. 5a ). As far as we know, such a rotation speed is the highest achieved in natural or man-made motors of the same scale. It is of the same speed level of jet engine, but is still not the limit. In comparison, the highest speed of nanomotors with bearings for position fixed rotation is 44.4–498 r.p.m., obtained from the organic–inorganic hybrid nanomotors [13] . 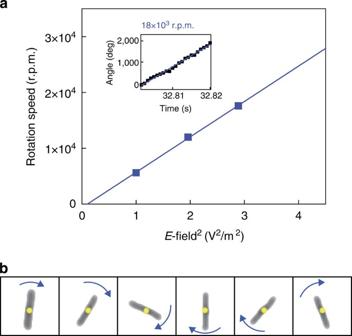Figure 5: Ultrahigh-speed rotation. (a) Rotation speed (ω) of nanomotors from 10 to 17 V at 30 kHz in a 100-μm-gapped quadruple microelectrode. (Inset) Angle (θ) versus time of the nanomotor rotating CW with a speed of ~18,000 r.p.m. (b) Enhanced snapshot images taken every 0.8 ms of the same nanomotor rotating at ~18,000 r.p.m. at 17 V and 30 kHz. Figure 5: Ultrahigh-speed rotation. ( a ) Rotation speed ( ω ) of nanomotors from 10 to 17 V at 30 kHz in a 100-μm-gapped quadruple microelectrode. (Inset) Angle ( θ ) versus time of the nanomotor rotating CW with a speed of ~18,000 r.p.m. ( b ) Enhanced snapshot images taken every 0.8 ms of the same nanomotor rotating at ~18,000 r.p.m. at 17 V and 30 kHz. Full size image Ultrasmall nanomotors One of the biggest advantages of nanomotors is their small footprint. No physical principles prevent rotation of even smaller motors. Using a microscope equipped with a × 100 oil-immersion objective and thin coverslips as substrates, we clearly observed controllable rotation of nanomotors made of three-segment nanowire rotors of 165 nm in diameter and 800–900 nm in total length (Au (350–400 nm)/Ni (100 nm)/Au (350–400 nm)) and magnetic bearings of 200 nm in diameter (made of tri-layer thin-film stack of Au (20 nm)/Ni (80 nm)/Cr (6 nm)) ( Fig. 6a–c ). All characteristic dimensions of the nanomotors are <1 μm, which is at least 10 times smaller than that of the state-of-the-art micromotors fabricated through the top-down approach. The nanomotors are even smaller than the motors made from nanotubes [12] . The nanomotor rotates in both CW and CCW directions at 15 V and 50 kHz as shown in Fig. 6d,e and Supplementary Movie 6 . The rotation speed is not as uniform as those of nanowire motors of a few micrometres in length, which can be attributed to stronger Brownian motions found in smaller objects in suspension. The ultimate size limit of nanomotors should be determined by Brownian motions, which is under investigation. We expect to be able to further decrease the length of the nanomotors, which requires new techniques to characterize their motions with optical microscopes. 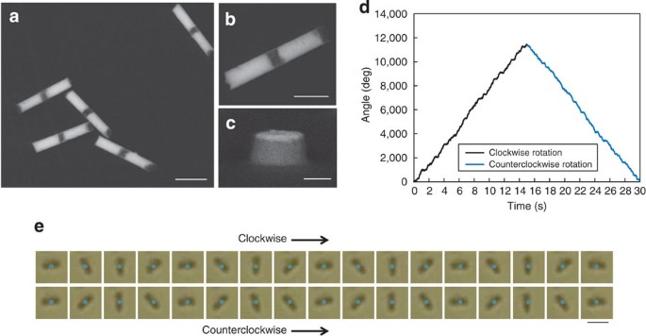Figure 6: Nanomotors with all dimensions <1 μm. (a) SEM images of the as-synthesized Au/Ni/Au nanowires (800–900 nm in length and 165 nm in diameter). Scale bar, 500 nm. The Au (bright) and Ni (dark) segments are 350–400 nm and 100 nm, respectively. (b) A close-up image of a single nanowire (scale bar, 300 nm). (c) Magnetic bearings of ~200 nm ((Au (20 nm)/Ni (80 nm)/Cr (6 nm) thin-film stacks) in diameter (scale bar, 100 nm). (d) Rotation angle as a function of time for both CW and CCW rotation of a nanomotor made of nanowires and magnetic bearings shown in (a–c). (e) Snapshots of a rotating nanomotor taken every 60 ms (the position of the magnetic bearing is highlighted with turquoise; scale bar is 1 μm). The real time rotation video is given in theSupplementary Movie 6. Figure 6: Nanomotors with all dimensions <1 μm. ( a ) SEM images of the as-synthesized Au/Ni/Au nanowires (800–900 nm in length and 165 nm in diameter). Scale bar, 500 nm. The Au (bright) and Ni (dark) segments are 350–400 nm and 100 nm, respectively. ( b ) A close-up image of a single nanowire (scale bar, 300 nm). ( c ) Magnetic bearings of ~200 nm ((Au (20 nm)/Ni (80 nm)/Cr (6 nm) thin-film stacks) in diameter (scale bar, 100 nm). ( d ) Rotation angle as a function of time for both CW and CCW rotation of a nanomotor made of nanowires and magnetic bearings shown in ( a – c ). ( e ) Snapshots of a rotating nanomotor taken every 60 ms (the position of the magnetic bearing is highlighted with turquoise; scale bar is 1 μm). The real time rotation video is given in the Supplementary Movie 6 . Full size image Durability of nanomotors How durable are these nanomotors? We performed a test to let the devices rotate without any interruption, and found that these nanomotors can keep rotating for up to 15 h ( Supplementary Movie 7 ), which results in >240,000 cycles in total ( Fig. 7a ). To our best knowledge, this is a record in both duration time and number of cycles among all reported rotary motors made from synthesized nanoparticles. This performance has surpassed the recent top-down-made Si micromotors [11] , showing the realistic potential of our nanomotors. After 15 h rotation, the Au cap layer on magnetic bearing was significantly thinned by frictional wearing. The scanning electron microscope (SEM) image in Fig. 7c reveals the final Au thickness of ~15 nm, reduced from its original thickness of 40 nm ( Fig. 7b,c ). No clear wear was found on the nanowire rotor ( Fig. 7c ), which can be attributed to the fact that Au (Vickers hardness: 216 MPa) is much softer than Ni (Vickers hardness: 638 MPa). The rotation of nanomotors was finally terminated by the increased magnetic attraction force and the consequential larger friction between rotors and bearings because of the reduced thickness of the Au layer resulted from frictional wearing. 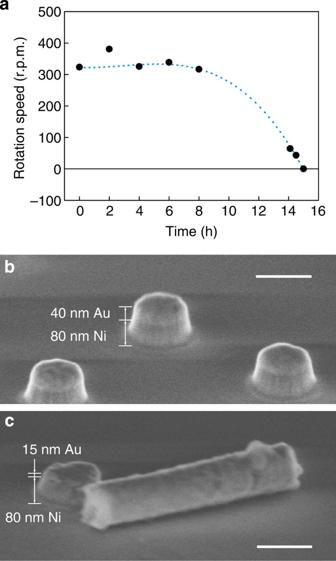Figure 7: Fifteen hours continuous rotation. Nanomotors (rotor: Au (350–400 nm)/Ni(100 nm)/Au(300–400 nm), 165 nm in diameter; bearing: ~200 nm in diameter, thin-film stack of Au (40 nm)/Ni (80 nm)/Cr (6 nm)) can be rotated continuously for up to 15 h. (a) Rotation speed versus time at 15 V and 30 kHz ACE-fields. Experimental data is presented as the black dots with the blue dotted trend line. (b) SEM images of the as-fabricated-magnetic bearings. (c) SEM images of the magnetic bearing and nanowire rotor after 15-hour rotation. Scale bars, 200 nm. Figure 7: Fifteen hours continuous rotation. Nanomotors (rotor: Au (350–400 nm)/Ni(100 nm)/Au(300–400 nm), 165 nm in diameter; bearing: ~200 nm in diameter, thin-film stack of Au (40 nm)/Ni (80 nm)/Cr (6 nm)) can be rotated continuously for up to 15 h. ( a ) Rotation speed versus time at 15 V and 30 kHz AC E -fields. Experimental data is presented as the black dots with the blue dotted trend line. ( b ) SEM images of the as-fabricated-magnetic bearings. ( c ) SEM images of the magnetic bearing and nanowire rotor after 15-hour rotation. Scale bars, 200 nm. Full size image Controlled biochemical release from nanomotors Finally, the applications of nanowire motors were demonstrated for rotation-controlled biochemical release as shown in Fig. 8a . In this study, we chose Nile blue molecules to demonstrate controllable molecular release by mechanically rotating nanomotors, considering their large Raman scattering cross-sections for optical characterization and wide usage in tagging biomolecules for biological study. By functionalizing the surface of nanowire rotors with surface-enhanced Raman scattering (SERS)-sensitive Ag nanoparticles ( Supplementary Note 4 ) [38] , we detected time-dependent release of Nile blue molecules from single rotating nanomotors using Raman spectroscopy ( Supplementary Movie 8 ). The release rate ( k ) monotonically increases with the rotation speeds of nanomotors ( Fig. 8b ; Supplementary Fig. 5 and Supplementary Note 5 ). Biochemical release from nanoparticles can be controlled predictably by mechanical rotation, which is a completely new actuation mechanism for biochemical release [39] . The fundamental principle can be attributed to thickness change of stationary diffusion layers, which will be studied elsewhere. Such molecule release mechanism is applicable not only to Raman-sensitive molecules but also to any biochemicals of interests, such as drugs, cytokine, DNA, antigens and antibodies. 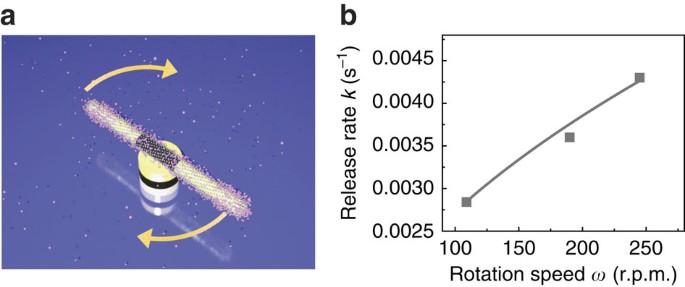Figure 8: Controlled biochemical release by nanomotors. (a) Illustration of rotation controlled release of biochemicals (the motor fixed on the nanomagnet is surface-enhanced Raman scattering (SERS) sensitive, which is a silica-shelled Au–Ni–Au nanowire with uniform surface distributed Ag nanoparticles). The nanomotor is functionalized with Nile blue (in pink). (b) The release ratekmonotonically increases with the rotation speeds of nanomotors. Figure 8: Controlled biochemical release by nanomotors. ( a ) Illustration of rotation controlled release of biochemicals (the motor fixed on the nanomagnet is surface-enhanced Raman scattering (SERS) sensitive, which is a silica-shelled Au–Ni–Au nanowire with uniform surface distributed Ag nanoparticles). The nanomotor is functionalized with Nile blue (in pink). ( b ) The release rate k monotonically increases with the rotation speeds of nanomotors. Full size image The demonstration of nanomotors for biochemical release as shown above is still in a non-bioenvironment. More experiments are necessary to study the applications and limitations of nanomotors in a biosetting. It will also be interesting to exam the release characteristics from multiple nanomotors. In our previous work, we successfully used electric tweezers to deliver drug functionalized nanowires to a single live cell amidst many and characterized responses from the cell [5] , which proved the compatibility of electric tweezers with the actual bioenvironment [5] . Here, the assembling and actuation of nanomotors in a biosetting should be also feasible, as the same electric tweezers technique is used. We envision the nanomotors as a unique tool for tunable release of biochemicals to a single live cell, which is important for understanding the fundamental signal transduction on single-cell levels [5] . One of the foreseen difficulties is how to position magnetic bearings in the vicinity of selected live cells for assembling nanomotors. This obstacle could be overcome by fabricating magnetic nanobearings on a wafer scale as shown in Supplementary Fig. 6 . Growing cells (typically 10 μm) on such substrates and controlling the density of the magnetic bearings, one can always find a few magnetic bearings close to a live cell for nanomotor assembling. We note that more work should be conducted to optimize the conditions, that is, the amount of chemicals loaded on the nanomotors and the control of distance of the nanomotors to the cell. Various biochemicals of interests apart from Nile blue should be tested. Also note that the nanomotors can release chemicals to the vicinity of cells, whereas cannot deliver chemicals into cells as shown by other reports. The materials used for nanomotors should be carefully selected. Non-biocompatible materials, such as Ni in nanowires and magnetic bearings, should be replaced with biocompatible magnetic materials, such as iron, or covered with materials innocuous to cells and bio molecules. Also, the method described above is suitable for single/few cell study in an i n vitro setting. It is not applicable to in vivo study. In terms of in vivo applications, in this work, we found that the release rate of biochemicals can be controlled by mechanically rotating nanoparticles. If we want to control the release rate of chemicals delivered into a human body by nanoparticles, we should directly rotate those nanoparticles in vivo by remotely applied electromagnetic fields. The integration of nanoparticles to a desired organism could be realized by the well-established site-specific bioconjugation technique [40] . A high-frequency AC field could be generated at a specific position by an endoscope-like device. All of these require extensive and careful investigation; especially the biocompatibility of high frequency E-fields of tens of kHz with a live organism is unknown. Overall, we demonstrated tunable biochemical release using nanomotors in a simple aqueous environment. Further experiments as discussed above are our next work to explore its usage in actual biosetting. If successful, the tunable release of biochemicals from nanomotors could be potentially pivotal for study of single-cell stimulation, cell–cell communication, system biology and drug delivery. In summary, we demonstrated innovative design, assembling and actuation of rotary NEMS devices using a strategic bottom-up nanoassembly and manipulation technique, the electric tweezers, which was reported previously. Ordered arrays of nanomotors can be efficiently assembled and synchronously rotated with controlled angle, speed and chirality. The rotation speed can be at least 18,000 r.p.m., which is still not the limit. Various complex nanoscale forces and torques involved in the nanomotor system are quantitatively modelled and determined, which is critical for understanding, design and actuation of various metallic NEMS devices. The nanomotors, with all dimensions <1 μm, can rotate continuously up to 15 h for more than 240,000 cycles. They were demonstrated for controlled biochemical release in a simple non-biosetting, and presented a new mechanical approach for tuning releasing rate of biochemicals from nanoparticles. The innovations reported in this research could be of interest for NEMS, bioNEMS, microfluidics and lab-on-a-chip architectures. Fabrication of nanowires In a three-electrode setup, Cu layer on the back of nanoporous anodized aluminium oxide template, Pt mesh and a Ag/AgCl electrode serve as a working electrode, a counter electrode and a reference electrode, respectively. The growth of the nanowires commences at the bottom of nanopores at the working electrode. The amount of electric charges passing through the circuit controls the length of each segment. As a result, arrays of nanowires, with a structure of 100–1,000-nm-long Ni segment sandwiched between two 350–500-nm-long Au segments were synthesized and suspended in DI water. Creation of rotating E-fields Rotating AC E -fields can be generated in the centre of quadruple microelectrodes by applying four AC voltages with 90° sequential phase shifts on the four sub-electrodes [41] . How to cite this article: Kim, K. et al . Ultrahigh-speed rotating nanoelectromechanical system devices assembled from nanoscale building blocks. Nat. Commun. 5:3632 doi: 10.1038/ncomms4632 (2014).